A strong bimetal-support interaction in ethanol steam reforming The metal-support interaction (MSI) in heterogeneous catalysts plays a crucial role in reforming reaction to produce renewable hydrogen, but conventional objects are limited to single metal and support. Herein, we report a type of RhNi/TiO 2 catalysts with tunable RhNi-TiO 2 strong bimetal-support interaction (SBMSI) derived from structure topological transformation of RhNiTi-layered double hydroxides (RhNiTi-LDHs) precursors. The resulting 0.5RhNi/TiO 2 catalyst (with 0.5 wt .% Rh) exhibits extraordinary catalytic performance toward ethanol steam reforming (ESR) reaction with a H 2 yield of 61.7%, a H 2 production rate of 12.2 L h −1 g cat −1 and a high operational stability (300 h), which is preponderant to the state-of-the-art catalysts. By virtue of synergistic catalysis of multifunctional interface structure (Rh-Ni δ − -O v -Ti 3+ ; O v denotes oxygen vacancy), the generation of formate intermediate (the rate-determining step in ESR reaction) from steam reforming of CO and CH x is significantly promoted on 0.5RhNi/TiO 2 catalyst, accounting for its ultra-high H 2 production. Supported metal catalysts with metal-support interaction (MSI) have been widely demonstrated in heterogeneous catalysis for many industrially important reactions (e.g., hydrogenation, oxidation, and catalytic reforming) [1] , [2] , [3] . Especially, the strong metal-support interaction (SMSI), a term to describe the phenomenon that the geometric and electronic structure of metal species is modified through interaction with supports has attracted considerable research interest for decades. More recently, Bao, Zhang, de Jong, and Christopher et al. reported a number of new strategies to regulate SMSI including redox-regulated (Pt/TiO 2 , Co/ Nb 2 O 5 ) [4] , [5] , particle size-controlled (Ir/CeO 2 , Ru/TiO 2 ) [6] , [7] , adsorbate-mediated (Ni/TiO 2 , Ru@MoO 3− x , and Rh/Nb 2 O 5 ) [8] , [9] , soft/wet chemistry-assisted (Au@TiO 2 ) [10] , [11] and crystal phase/facet-guided catalysts (Ru/TiO 2 and Pd/TiO 2 ) [12] , [13] . In these cases, effective supports with engineered characteristics have been successfully employed to stabilize metal species, modify its geometric/electronic structure, and regulate mass transfer efficiency. Importantly, the proximity of active metal species to support defects also makes a great contribution to promote the activation adsorption of reactants, optimize the transition state of adsorbates and facilitate the transformation of reaction intermediates [14] , [15] , [16] . In general, the SMSI involved in heterogeneous metal catalysts plays a critical role in boosting catalytic performance toward structure-sensitive reactions. Hydrogen (H 2 ) with a high energy density and zero pollution is being contemplated as the most promising alternative energy, which has been globally explored based on steam reforming of hydrocarbons and oxygenates (e.g., CH 4 , CO, CH 3 OH, and CH 3 CH 2 OH) in the preceding decades [3] , [17] , [18] , [19] , [20] , [21] , [22] , [23] , [24] , [25] , [26] , [27] , [28] , [29] . Ethanol, with low toxicity and high hydrogen/carbon ratio, which can be facilely produced from renewable biomass, has been employed as a hydrogen feedstock through ethanol steam reforming (ESR) reaction [18] , [24] , [25] , [26] , [27] , [28] , [29] . In respect to such a structure-sensitive reaction, the metal active sites are geometrically and electronically modified via SMSI, and the supports in most cases participate in the catalytic reaction [2] , [15] . Nevertheless, the conventionally reported SMSI is normally focused on individual metal and oxide support, whose single-channel interaction shows restriction when applied in certain complex processes [4] , [16] , such as ESR reaction involving multiple sequential steps. Therefore, how to develop sophisticated catalysts based on multichannel SMSI with largely enhanced catalytic performance for ESR still remains a huge challenge. Meanwhile, an in-depth insight into interfacial active sites at the atomic level is crucial for understanding reaction mechanism and pathway. In this work, we prepared a series of x RhNi/TiO 2 catalysts with tunable strong bimetal-support interactions (SBMSI) based on a topotactic transformation from RhNiTi-layered double hydroxides (RhNiTi-LDHs) precursors. The CO-DRIFT and STEM confirm the existence of a significantly reversible TiO 2 coating over RhNi bimetallic nanoparticle. The coordination and electronic structure between RhNi bimetal and TiO 2 support are facilely regulated via changing the doping content of Rh, which realizes a multi-transfer pathway of electrons and further optimizes the interfacial active sites (Rh-Ni δ − -O v -Ti 3+ ). The resulting 0.5RhNi/TiO 2 (with 0.5 wt .% Rh) sample exhibits a prominent catalytic performance toward ESR reaction, with an ethanol conversion of 99.7% and a H 2 yield of 61.7% at 400 °C. The H 2 production rate reaches 12.2 L h −1 g cat −1 with an outstanding catalysis stability within 300 h, which is preponderant to the state-of-the-art catalysts. The steam reforming of CO and CH x , which is the crucial step affecting H 2 production in ESR, is largely boosted at the interfacial sites (Rh-Ni δ − -O v -Ti 3+ ). Kinetic studies combined with in situ characterizations (XAFS and FT-IR) and DFT theoretical calculations demonstrate that the SBMSI in 0.5RhNi/TiO 2 catalyst not only promotes the formation of formate intermediate (the rate-determining step), but also alleviates the strong binding of formate and CO 2 on catalyst surface, both of which are beneficial to the transformation of reactants and the regeneration of active sites. Synthesis and characterization of x RhNi/TiO 2 catalysts The XRD patterns show a series of typical characteristic diffraction peaks of hydrotalcite-like structure (003, 006, 012, and 110) in as-synthesized x RhNiTi-LDHs precursors (Supplementary Fig. 1a ). As shown in the SEM images (Supplementary Fig. S2 ), the introduction of trace Rh does not significantly affect its surface topography, and all these samples display a frizzy flowerlike morphology. After a treatment in H 2 atmosphere at 400 °C, the crystallite surface becomes rough with enhanced specific surface area and enriched pore structure (Supplementary Fig. 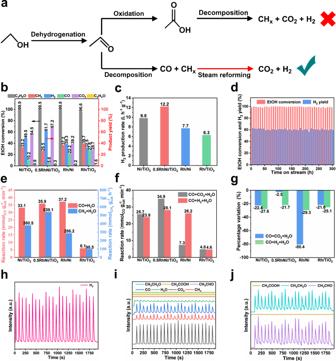Fig. 1: Catalytic performance toward ESR reaction and kinetic studies on CO and CH4reforming. aSchematic representation for the reaction paths of ESR reaction (Red arrow indicates the key step).bEthanol conversion, products yield andcH2production rate over various catalysts (reaction conditions: catalyst (0.15 g) + SiO2(1.50 g); liquid feed of S/C = 3 at 0.060 mL min−1; N2carrier at 50.0 mL min−1; reaction temperature: 400 °C; time on stream: 1.5 h).dTime on stream (TOS) test of 0.5RhNi/TiO2catalyst at 400 °C.e,fReaction rate for CO/CH4steam reforming reaction within kinetic range (CO or CH4conversion <10%). Reaction conditions: catalyst (5 mg) + SiO2(50 mg), liquid feed of H2O at 0.032 mL min−1, CO at 50.0 mL min−1, CH4at 10 mL min−1, CO2/H2at 10.0 mL min−1, N2carrier at 50 mL min−1, reaction temperature: 400 °C, time on stream: 0.5 h.gPercentage variation in reaction rate of CO steam reforming with CO2/H2addition over Ni/TiO2, 0.5RhNi/TiO2, Rh/Ni, and Rh/TiO2catalysts, respectively.h,iMS signals from theoperandopulse experiment of ethanol and water (S/C = 3) over 0.5RhNi/TiO2catalyst at 400 °C.jEnlarged view for MS signals of the three species ini. 3 and Supplementary Table 1 ). The crystal structure of as-obtained x RhNi/TiO 2 samples is indexed to a superimposition of face-centered cubic (fcc) Ni (JCPDS 7440-02-0) and anatase TiO 2 phase (JCPDS 21-1272) (Supplementary Fig. 1b ). Transmission electron microscopy (TEM) and high-resolution transmission electron microscope (HR-TEM) images of x RhNi/TiO 2 samples show that Ni nanoparticles (particle size: 12−16 nm) are uniformly dispersed within the TiO 2– x matrix (Supplementary Figs. 4 and 5 ). Especially, a well-defined metal-support (Ni-TiO 2 ) interface structure is clearly observed in these x RhNi/TiO 2 samples (Supplementary Fig. 5 and Supplementary Note 1 ). Catalytic performance and kinetic analysis toward ESR The ESR reaction was performed in a fixed-bed reactor with steam/carbon (S/C) ratio of 3. Compared with Ni/TiO 2 and Rh/TiO 2 , the RhNi/TiO 2 and Rh/Ni catalysts remarkably promote the conversion of ethanol and acetaldehyde at 350 °C (Supplementary Figs. 6a, b ), indicating the advantages of RhNi bimetal system. As the reaction temperature reaches 400 °C, an almost complete conversion of ethanol and acetaldehyde is obtained for all these catalysts, but the distribution of gas product (CO, CO 2 , CH 4 , and H 2 ) is significantly different (Fig. 1b and Supplementary Fig. 6c ). This indicates that the cleavage of C−C, O−H and C−H bonds in ethanol and acetaldehyde is sensitive to reaction temperature, and 400 °C is required for the breakage of the chemical bonds above. For the x RhNi/TiO 2 catalysts, the H 2 yield shows a volcanic trend as Rh content increases from 0 to 1%, and the maximum value is present in 0.5RhNi/TiO 2 sample (H 2 yield: 61.7%; production rate: 12.2 L h −1 g −1 ) (Fig. 1c and Supplementary Fig. 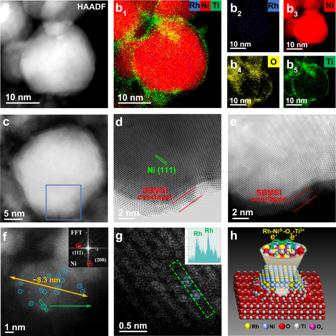Fig. 2: Microstructure fine-structure characterizations. a,c,dac-HAADF-STEM andeBF-STEM images,b1–b5corresponding EDS mapping, andf,ghigh-resolution STEM images of the 0.5RhNi/TiO2catalyst with atomically dispersed Rh species marked by blue circles.hSchematic diagram of the 0.5RhNi/TiO2catalyst. 7 ), which is preponderant to the state-of-the-art catalysts for ESR (Supplementary Table 2 ). Furthermore, we also tested the ESR reaction at a higher WHSV (21 h −1 ) and GHSV (16700 h −1 ) at 400 °C (ethanol conversion less than 70%), and the 0.5RhNi/TiO 2 catalyst still displayed the optimal hydrogen yield and relatively low CH 4 and CO yields (Supplementary Fig. 8 ). This is in sharp contrast to the Rh/NiO and Rh/TiO 2 samples, which give a much lower H 2 yield but a higher proportion of CO and CH 4 species (Fig. 1b ), showing the superiority of bimetal-support (RhNi-TiO 2 ) system. In addition, the time on stream (TOS) tests for Ni/TiO 2 , Rh/Ni, Rh/TiO 2 , and 0.5RhNi/TiO 2 were carried out at 400 °C, respectively. After the reaction for 40 h, the ethanol conversion over Ni/TiO 2 , Rh/Ni, and Rh/TiO 2 decreases from 100% to 91.33%, 58.54%, and 74.16%, respectively (Supplementary Fig. 9 ). In contrast, both the ethanol conversion and hydrogen yield in the presence of 0.5RhNi/TiO 2 catalyst remain stable within 300 h (Fig. 1d ). The crystal structure and particle size of the used catalyst do not show obvious change except for the formation of certain carbon-accumulating species (Supplementary Fig. 10 ). Fig. 1: Catalytic performance toward ESR reaction and kinetic studies on CO and CH 4 reforming. a Schematic representation for the reaction paths of ESR reaction (Red arrow indicates the key step). b Ethanol conversion, products yield and c H 2 production rate over various catalysts (reaction conditions: catalyst (0.15 g) + SiO 2 (1.50 g); liquid feed of S/C = 3 at 0.060 mL min −1 ; N 2 carrier at 50.0 mL min −1 ; reaction temperature: 400 °C; time on stream: 1.5 h). d Time on stream (TOS) test of 0.5RhNi/TiO 2 catalyst at 400 °C. e , f Reaction rate for CO/CH 4 steam reforming reaction within kinetic range (CO or CH 4 conversion <10%). Reaction conditions: catalyst (5 mg) + SiO 2 (50 mg), liquid feed of H 2 O at 0.032 mL min −1 , CO at 50.0 mL min −1 , CH 4 at 10 mL min −1 , CO 2 /H 2 at 10.0 mL min −1 , N 2 carrier at 50 mL min −1 , reaction temperature: 400 °C, time on stream: 0.5 h. g Percentage variation in reaction rate of CO steam reforming with CO 2 /H 2 addition over Ni/TiO 2 , 0.5RhNi/TiO 2 , Rh/Ni, and Rh/TiO 2 catalysts, respectively. h , i MS signals from the operando pulse experiment of ethanol and water (S/C = 3) over 0.5RhNi/TiO 2 catalyst at 400 °C. j Enlarged view for MS signals of the three species in i . Full size image The operando infrared spectra (Supplementary Figs. 11 – 13 and Supplementary Note 2 ) were performed to identify the ESR reaction path. The results from the infrared spectra verify that the ESR reaction over 0.5RhNi/TiO 2 , Ni/TiO 2 , and Rh/Ni catalysts undergoes ethanol dehydrogenation to acetaldehyde followed by acetaldehyde decomposition to CO and CH x (CO/CH x -mediated reforming process), rather than the acetate paths (Fig. 1a ) [24] , [28] , [29] . The resulting CO and CH x as key intermediates continue to react with H 2 O to produce CO 2 and H 2 . This is consistent with the results from the operando pulse experiment of ethanol and water (Fig. 1h–j ) with mass spectrometer (MS), where the characteristic bands assigned to various reaction intermediates are observed whilst acetate species are not detected during the whole reaction process. Thus, the H 2 yield depends heavily on the transformation of these CO and CH x intermediates, in addition to ethanol conversion. Furthermore, we performed kinetic tests on ethanol dehydrogenation, acetaldehyde decomposition, steam reforming of CO (or CH 4 ) to study the C−H bond cleavage, C−C bond cleavage, CO or CH x transformation during ESR reaction. As shown in Supplementary Fig. 14a , the apparent activation energy of these reaction processes gives the following sequence: ethanol dehydrogenation (44.54 kJ mol −1 ) < acetaldehyde decomposition (50.45 kJ mol −1 ) < CO steam reforming (89.46 kJ mol −1 ) < CH 4 steam reforming (101.26 kJ mol −1 ), which indicates that the cleavage of C−H and C−C bonds in ethanol is facile whilst the transformation of intermediates (CO and CH x ) is rather difficult. This result is further demonstrated through a more significantly concentration-dependent reaction order for CO and CH 4 in comparison with ethanol and acetaldehyde: ethanol (0.46) < acetaldehyde (0.62) < CO (1.18) < CH 4 (1.23) (Supplementary Fig. 14b ). In addition, we contrasted the conversion rates of CO and CH 4 over these samples (Fig. 1e ). The CO conversion declines in the following sequence: Rh/Ni > 0.5RhNiTi > NiTi >> Rh/TiO 2 ; whilst CH 4 conversion decreases in order: 0.5RhNiTi > NiTi > Rh/Ni > Rh/TiO 2 . The higher CO conversion rate on Rh/Ni is not consistent with its high CO yield. Considering that the reaction mixture would reach equilibrium at prolonged reaction time, and the products (H 2 and CO 2 ) may affect the progress of main reaction, we measured the reaction rate of water-gas shift (WGS) reaction by adding a small amount of H 2 or CO 2 into the reaction atmosphere (Fig. 1f ). A similar decrease extent is observed for these catalysts after H 2 introduction (Fig. 1g ), indicating that the inhibitory effect mainly originates from the equilibrium limit (Le Chatelier’s principle). In contrast, these catalysts show a significantly difference in CO reaction rate after CO 2 introduction: a remarkable decline ratio of 80.4% (from 37.2 to 7.3 mol CO g cat −1 min −1 ) is obtained over Rh/Ni catalyst, relative to 0.5RhNi/TiO 2 with a slight decrease of 2.5%, indicating the existence of other important factors besides equilibrium limit. Moreover, the CO 2 -TPD (Supplementary Fig. 15 and Supplementary Note 3 ) and reaction order measurements (Supplementary Fig. 16 and Supplementary Note 4 ) confirm that Rh/Ni catalyst shows a stronger CO 2 adsorption ability and a more negative CO 2 reaction order (−0.64) compared with 0.5RhNi/TiO 2 (−0.18), demonstrating a stronger inhibitory action by CO 2 in the former case. In addition, the conversion of CO and CH 4 are also determined when H 2 O, CO, CH 4 , H 2 , and CO 2 are present in the reactants simultaneously (Supplementary Fig. 17 and Supplementary Note 5 ), and 0.5RhNi/TiO 2 catalyst still exhibits the highest conversion of CH 4 and CO. Thus, the kinetic studies above substantiate that 0.5RhNi/TiO 2 catalyst possesses a powerful catalytic transformation ability toward CO and CH x as well as a strong resistance against CO 2 , resulting in its extraordinary catalytic performance toward ESR. Microstructure investigations and fine-structure characterizations Aberration-corrected high-angle annular dark-field scanning transmission electron microscopy (ac-HAADF-STEM) image and energy-dispersive spectroscopy (EDS) measurements were carried out to explore the interfacial structure of x RhNi/TiO 2 samples (Fig. 2 and Supplementary Figs. 18 – 23 ). For 0.3RhNi/TiO 2 and 0.5RhNi/TiO 2 catalysts, Rh tends to present an atomic-level dispersion on the surface of Ni particles to form RhNi bimetallic structure (Fig. 2f, g , and Supplementary Fig. 18 ), and a significant interface encapsulation of TiO 2 on the surrounding of RhNi nanoparticle is observed after H 2 activation (Fig. 2 b 1 –b 5 , d, e, and Supplementary Fig. 20 ). However, visible TiO 2- x overlayer recedes over RuNi bimetallic NPs when exposed to air oxidation conditions (Supplementary Fig. 21 ), which is consistent with the phenomenon from classical SMSI [4] , [9] , [13] , [16] , [30] , [31] , [32] . For 0.8RhNi/TiO 2 and 1.0RhNi/TiO 2 sample with a higher Rh content, Rh species shows an aggregation state on the surface of Ni particles (Supplementary Figs. 22 and 23 ). The results intuitively confirm the well-defined interface structure between RhNi bimetal and TiO 2 support. In addition, Ni/TiO 2 and Rh/TiO 2 samples also show classic SMSI effect as demonstrated by STEM and elemental line scanning, in which the reversible overlayer of TiO 2– x appears and disappears under the reduction and oxidation conditions, respectively (Supplementary Figs. 24 – 26 ). Fig. 2: Microstructure fine-structure characterizations. a , c , d ac-HAADF-STEM and e BF-STEM images, b 1 – b 5 corresponding EDS mapping, and f , g high-resolution STEM images of the 0.5RhNi/TiO 2 catalyst with atomically dispersed Rh species marked by blue circles. h Schematic diagram of the 0.5RhNi/TiO 2 catalyst. Full size image The CO-DRIFT was used to further identify the structure evolution as demonstrated above (Fig. 3a–c , and Supplementary Fig. 27 ). The peaks at 2115, 2104, and 2096 cm −1 are assigned to the CO adsorbed at Ni and Rh sites, and the bands at 2080 and 2046 cm −1 are attributed to RhNi bimetallic interface sites. The alternative changes of weakened and strengthened CO adsorption intensity during five-cycle of H 2 reduction-O 2 oxidation correspond to a reversible encapsulation and decapsulation of TiO 2- x overlayer. Notably, a more pronounced variation is observed over 0.5RhNi/TiO 2 catalyst, signifying a stronger interaction from RhNi bimetal and TiO 2 support. For Rh/Ni sample, the Rh clusters are dispersed on Ni without SMSI effect (Supplementary Figs. 27 and 28 ). Fig. 3: Geometric and electronic properties characterizations. CO-DRIFT spectra at ambiance temperature over a 0.5RhNi/TiO 2 , b Ni/TiO 2 , and c Rh/TiO 2 catalysts during five-cycle H 2 reduction-O 2 oxidation. XPS spectra of d Ni 2 p , e Ti 2 p , and f O 1 s for various samples. Normalized spectra of g Ni K-edge XANES, h Ni K-edge EXAFS at R-space, and i Ti K-edge XANES for various samples. Full size image The electronic structure of x RhNi/TiO 2 samples was investigated by X-ray photoelectron spectroscopy (XPS). As the Rh content increases from 0 to 0.5%, the binding energy of Ni 2 p moves to higher energy, indicating a decreased Ni electron density on 0.5RhNi/TiO 2 catalyst (Fig. 3d and Supplementary Note 6 ). However, with a further increase of Rh loading from 0.5% to 1.0%, the binding energy of Ni shifts back to lower energy. The binding energy of Rh exhibits an opposite variation relative to Ni (Supplementary Fig. 29 ). The results indicate that the electron transfer from Ni to Rh becomes weak when the Rh distribution converts from atomic level to clusters or particles. This volcanic change trend of electron density for Ni species verifies that this bimetal-support interface breaks through the traditional electron transfer mode between single metal and oxide support. Compared with Ni/TiO 2 , the Ti 3+ /(Ti 3+ +Ti 4+ ) ratio in x RhNi/TiO 2 samples declines gradually with the increment of Rh loading (Fig. 3e ). Notably, the Ti 3+ species in Rh/TiO 2 displays a significant reduction compared with Ni/TiO 2 , indicating Ti 3+ mainly originates from Ni-TiO 2– x interaction and the formation of RhNi bimetal would change such interaction. In addition, the O β /(O α + O β + O γ ) ratio (O α : lattice oxygen O 2− ; O β : chemisorbed oxygen O − 2 or O − ; O γ : other oxygen species including adsorbed water) shows a rise firstly and then a decline (Fig. 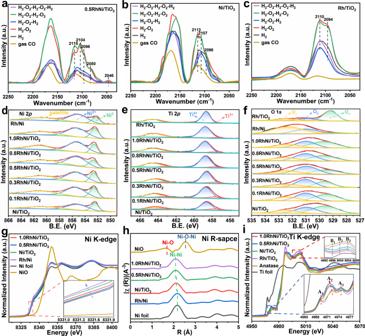Fig. 3: Geometric and electronic properties characterizations. CO-DRIFT spectra at ambiance temperature overa0.5RhNi/TiO2,bNi/TiO2, andcRh/TiO2catalysts during five-cycle H2reduction-O2oxidation. XPS spectra ofdNi 2p,eTi 2p, andfO 1sfor various samples. Normalized spectra ofgNi K-edge XANES,hNi K-edge EXAFS at R-space, andiTi K-edge XANES for various samples. 3f ), and the maximal value is present in 0.5RhNi/TiO 2 (Supplementary Table 3 ), indicating that a lower Ni electron density promotes the combination of oxygen species. The variation in RhNi-TiO 2 interaction was further proved by H 2 -TPR and H 2 -TPD analysis (Supplementary Fig. 30 and Supplementary Note 7 ). The results above demonstrate that the electronic effect in x RhNi/TiO 2 samples can be finely regulated through tuning Rh content. In addition, the interface electronic and coordination structure were studied via X-ray absorption spectroscopy (XAS). As shown in normalized XANES spectra of Ni K-edge (Fig. 3g ), the absorption edge of all samples is located at lower photon energy relative to Ni foil, indicating the existence of a negative valence state (Ni δ − species), which is similar to other TiO 2 -supported group VIII metals with electron transfer from TiO 2– x to the interfacial metal atoms [4] , [9] , [16] , [30] , [31] , [32] . Notably, the absorption edge of 0.5RhNi/TiO 2 displays a minimum shift to lower energy among these samples, indicative of the lowest electron density of interfacial Ni atom. Meanwhile, the fitting results from FT k 3 -weighted Fourier transforms of the extended X-ray absorption fine-structure (EXAFS) spectra and wavelet transforms (Fig. 3h , Supplementary Figs. 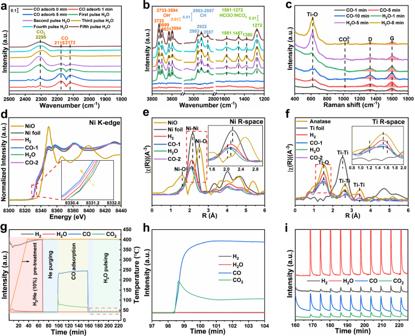Fig. 4: In situ characterizations and reaction mechanism of CO reforming. a,bIn situ DRIFT spectra,cin situ Raman spectra,din situ normalized XANES spectra,ein situ Fourier-transform EXAFS spectra at Ni K-edge in R-space, andfTi K-edge in R-space of CO adsorption and then H2O adsorption on 0.5RhNi/TiO2catalyst at 400 °C (H2, CO-1, H2O, and CO-2 denote the spectra after successive H2pretreatment, CO adsorption, H2O adsorption, and CO adsorption again for 20 min on 0.5RhNi/TiO2catalyst, respectively).gMass spectral analysis for CO and H2O pulse over 0.5RhNi/TiO2catalyst andh,icorresponding local magnification regions ing. 31 and 32 , and Supplementary Table 4 ) show that the Ni−Ni bond length in Ni/TiO 2 sample becomes shorter compared with Ni foil and Rh/Ni, owing to the interaction between Ni and TiO 2 support. Moreover, the Ni−Ni bond length in 0.5RhNi/TiO 2 and 1.0RhNi/TiO 2 shortens further relative to Ni/TiO 2 . The normalized Ti K-edge XANES data are presented in Fig. 3i . All the samples show similar curves to the anatase reference in pre-edge range (4968 to 4980 eV) and post-edge region (4992 to 5008 eV), but the A 1 peak and the three peaks (denoted as B 1 , B 2 and B 3 ) for Ni/TiO 2 , 0.5RhNi/TiO 2 and 1.0RhNi/TiO 2 samples are less resolved; and the intensity of their A 2 peaks becomes stronger accompanied with a shift to lower energy. The results indicate the presence of distorted octahedral Ti−O environment associated with oxygen vacancies [13] , [33] . Fourier transform of Ti K-edge EXAFS spectra display that the first shell of Ti−O bond in x RhNi/TiO 2 samples gives an obviously less than sixfold coordination number (Supplementary Fig. 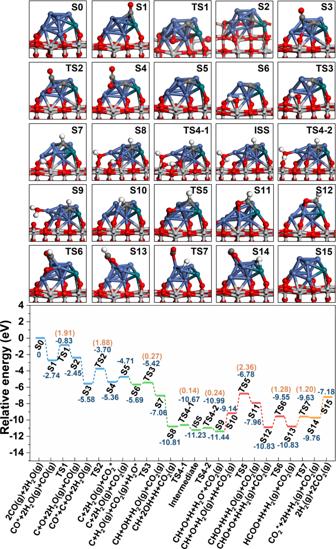Fig. 5: DFT calculation and schematic illustration. Reaction mechanism of stream reforming of CO on the surface of Rh1Ni7/TiO2–x. ‘S’ denotes a stable sorption state; ‘TS’ denotes a transition state; ‘ISS’ denotes an intermedia stable state. (Blue, green, red, and orange dotted lines indicate CO disproportionation, H2O dissociation, formate generation, and CO2desorption, respectively; blue and orange numbers represent adsorption energy and reaction energy barrier, respectively). 33 , Supplementary Table 5 and Supplementary Note 8 ), which is the most significant for 0.5RhNi/TiO 2 . Based on the results afore-mentioned, a unique geometric and electronic structure between RhNi bimetal and TiO 2 support in x RhNi/TiO 2 catalysts is demonstrated clearly (Fig. 2h ), defined as the strong bimetallic-support interaction (SBMSI), which is responsible for the outstanding catalytic performance of 0.5RhNi/TiO 2 . In situ spectral characterization for reaction mechanism Based on the catalytic evaluations and kinetic studies, the key steps determining H 2 generation is the transformation of intermediate products (CO and CH x ). A series of in situ DRIFT measurements were carried out to investigate the influence of SBMSI on CO and CH x transformation. As 0.5RhNi/TiO 2 is exposed to CO at 400 °C, CO 2 adsorption bands within 2270–2389 cm −1 appear [34] , [35] , whose intensity enhances gradually along with time, indicating the occurrence of CO disproportionation on the catalyst surface to produce CO 2 and C species (Supplementary Fig. 34 and Supplementary Note 9 ). Subsequently, a switching to H 2 O pulse leads to the decline of CO signal, accompanied by the formation of Ti 3+ −OH and Ti 4+ −OH species (3733–3594 cm −1 ); and several absorption bands including formate species (2953–2857, 1581, and 1380 cm −1 ) and bidentate hydrogen-carbonates species (1457 and 1272 cm −1 ) are observed (Fig. 4a, b ) [1] , [9] , [36] , [37] . The peak intensity of formate enhances firstly and then declines with the pulse of water, indicating that such species is an important reaction intermediate. To further identify the generation path for formate intermediate, another H 2 O pulse test is implemented again after purging the surface CO and CO 2 by He (Supplementary Fig. 35 ). The analogous formate intermediate is detected, indicating that formate is derived from the further transformation of carbon species produced by CO disproportionation. In situ Raman was further used to verify this issue (Fig. 4c ), in which two remarkable bands at 1330 and 1609 cm −1 ascribed to D and G bands of carbon species were observed after purging CO [18] , [38] , [39] . Afterwards, the band intensity of carbon species declines, and the Ti−O signal increases for 0.5RhNi/TiO 2 catalyst with the introduction of saturated water vapor. Furthermore, when CO and saturated water vapor are introduced together, very few carbon species are detected, indicating that accumulation and consumption of carbon maintain a balance under WGS reaction conditions (Supplementary Fig. 36 ). Fig. 4: In situ characterizations and reaction mechanism of CO reforming. a , b In situ DRIFT spectra, c in situ Raman spectra, d in situ normalized XANES spectra, e in situ Fourier-transform EXAFS spectra at Ni K-edge in R-space, and f Ti K-edge in R-space of CO adsorption and then H 2 O adsorption on 0.5RhNi/TiO 2 catalyst at 400 °C (H 2 , CO-1, H 2 O, and CO-2 denote the spectra after successive H 2 pretreatment, CO adsorption, H 2 O adsorption, and CO adsorption again for 20 min on 0.5RhNi/TiO 2 catalyst, respectively). g Mass spectral analysis for CO and H 2 O pulse over 0.5RhNi/TiO 2 catalyst and h , i corresponding local magnification regions in g . Full size image Furthermore, the TPSR-mass spectral analysis is carried out. Firstly, the 0.5RhNi/TiO 2 catalyst was pretreated in H 2 at 400 °C for 30 min followed by He flushing for 30 min. Then, the gas was switched to CO, He, and saturated water vapor in turn to monitor the gas signals (Fig. 4g–i ). The formation of CO 2 was detected synchronously with the introduction of CO, indicating the occurrence of CO disproportionation to generate CO 2 and C species (Fig. 4h ), in accordance with the results of in situ DRIFT (Fig. 4a and Supplementary Figs. 34 and 35a ) and in situ Raman spectra (Fig. 4c ). Subsequently, He flushing followed by a saturated water vapor pulse over the catalyst gave rise to the generation of H 2 and CO 2 (Fig. 4i ). Such phenomenon demonstrates that H 2 O dissociation occurs on oxygen vacancy of TiO 2 to generate active hydroxyl/oxygen groups, which further react with surface carbon species to give formate intermediate; subsequently, formate species undergoes decomposition to produce CO 2 and H 2 . The results above demonstrate that the WGS reaction obeys an associative mechanism on the surface of 0.5RhNi/TiO 2 . For Ni/TiO 2 catalyst, a similar associative reaction mechanism was also verified (Supplementary Figs. 38a and 39 ), except a lower intensity of formate intermediate, corresponding to its lower CO conversion (Supplementary Note 11 and Supplementary Note 12 ). For Rh/Ni catalyst without SBMSI, CO disproportionation process occurs; however, no associative reaction intermediate is detected after purging H 2 O pulse as proved by in situ DRIFT and in situ Raman results (Supplementary Fig. 40 and Supplementary Note 13 ). Furthermore, the mass spectral analysis confirms that H 2 O experiences dissociation over Rh/Ni catalyst to produce H 2 and active O species, and then O species reacts with CO or C species to form CO 2 (Supplementary Fig. 37 and Supplementary Note 10 ), which accords with redox mechanism [20] , [40] , [41] , [42] . Moreover, in situ Raman spectra also confirm the existence of carbonate species (1000−1200 cm −1 ) on Rh/Ni and 0.5RhNi/TiO 2 catalyst. The more significant intensity in the former case originates from a stronger binding of CO 2 (Fig. 4c and Supplementary Fig. 40c ), which is consistent with the test results. The impact of CO 2 was discussed in detail based on in situ DRIFT, in situ Raman and Quasi -in situ XPS in supporting information (Supplementary Figs. 41 – 44 and Supplementary Notes 14– 16 ), where 0.5RhNi/TiO 2 with SBMSI shows the strongest CO 2 resistance. For Rh/TiO 2 catalyst, CO disproportionation does not occur along with fewer reaction intermediates after H 2 O pulse (Supplementary Figs. 38c and 45 , and Supplementary Note 17 ), which is associated with its poor WGS reaction activity. In addition, we also carried out in situ DRIFT investigations for CH 4 steam reforming on these catalysts to imitate the transformation of CH x species. After purging CH 4 , an obvious peak appears at 1542 cm −1 assigned to bidentate formate intermediate on 0.5RhNi/TiO 2 , Ni/TiO 2 and Rh/Ni samples (Supplementary Fig. 46 ). When introducing saturated water vapor into the reaction cell at 400 °C, formate intermediate declines accompanied with the formation of CO 2 . Both the consumption rate of formate intermediate and the band intensity of δ (CH x ) at 1542 and 1302 cm −1 decrease in the following order: 0.5RhNi/TiO 2 > Ni/TiO 2 > Rh/Ni (Supplementary Fig. 47 and Supplementary Note 18 ), in accordance with the test results (Fig. 1b, e ). However, no obvious intermediate is found in the case of Rh/TiO 2 due to its poor catalytic performance (Supplementary Fig. 46h ). Furthermore, no obvious carbon species is observed in in situ Raman spectra for 0.5RhNi/TiO 2 and Rh/Ni catalysts, ruling out the complete dehydrogenation of CH x in reforming processes (Supplementary Fig. 48 and Supplementary Notes 19 ), since the most stable CH fragment can react with hydroxy group or active oxygen to produce formate intermediate (CH x → CH + H x –1 → HCOO − ) [37] , [43] , [44] , [45] . After switching to a saturated water vapor, carbonate species (1000−1200 cm −1 ) resulting from CO 2 behaves a stronger binding onto Rh/Ni than 0.5RhNi/TiO 2 catalyst (Supplementary Fig. 48 ), similar to the CO reforming process. Owing to the similar O−C−O structure of formate to CO 2 or carbonate, the lower conversion of CH x on Rh/Ni is possibly associated with the stronger binding of formate to Ni sites, which inhibits its further transformation. Therefore, the 0.5RhNi/TiO 2 catalyst with unique coordination and electronic structure resulting from SBMSI reduces the binding ability of species with analogous COO − structure (CO 2 , carbonate, or formate), and thus promotes the generation and transformation of formate intermediate, accounting for its excellent reforming activity of CO and CH x . In situ XAFS measurements were performed to track the dynamic evolution of coordination structure and electronic state of bimetal-support interface sites during steam reforming process. For the 0.5RhNi/TiO 2 sample, when CO is introduced into the reaction system (CO-1), the absorption edge of Ni shifts to lower energy (Fig. 4d ), accompanied with a decrease in the coordination number of Ni−Ni bond (Fig. 4e , Supplementary Fig. 49b and Supplementary Table 6 ). The corresponding variations in Ti K-edge XAFS spectra are also observed, where the A 2 peak shifts to lower energy (Supplementary Fig. 49c ) with a decline in the coordination number of Ti−O bond (Fig. 4f ). This is attributed to the catalyst reconstruction resulting from CO disproportionation, in which the generated carbon species fixed to Ni sites reacts with active oxygen species offered by TiO 2 at interface sites. Once the reaction atmosphere is switched to a saturated water vapor (H 2 O), the absorption edge of Ni moves toward higher energy and Ni−Ni bond length becomes shorter (Fig. 4d, e ), due to the formation of formate intermediate on the catalyst surface. In addition, the intensity of A 2 peak in Ti K-edge XANES spectra (Supplementary Fig. 49c ) declines and the Ti−O bond splits upon exposure to H 2 O vapor (Fig. 4f ). This is ascribed to the quenching of oxygen vacancy in TiO 2 by active hydroxy species (from Ti 3+ –O v to Ti 4+ –OH − ), along with a structure reconfiguration. After purging CO again (CO-2), the catalyst structure is restored to its original state and a reaction cycle is completed. The results substantiate that the bimetal-support interfacial sites participate in the steam reforming processes, accompanied by the interface reconstruction in the case of 0.5RhNi/TiO 2 catalyst. In contrast, the metal sites on Rh/Ni catalyst play a dual role toward activation adsorption of both water molecule and reactants, corresponding to its poor catalytic properties. A detailed discussion on in situ XAFS measurements was offered in supplementary materials (Supplementary Fig. 50 , Supplementary Table 7 and Supplementary Note 20 ). Furthermore, we carried out first-principle calculations to further understand the roles of bimetal-support interfacial sites in ethanol conversion and steam reforming processes of CO and CH x , and the Rh 1 Ni 7 /TiO 2- x model systems was built (Supplementary Fig. 51 and Supplementary Note 21 ). Based on the Bader charge analysis results, compared with the Ni 8 /TiO 2 -x (Supplementary Figs. 52a, c ), the Rh 1 Ni 7 /TiO 2 -x system (Supplementary Figs. 52b, d ) with SBMSI weakens the charge transfer from the oxygen vacancy on TiO 2 -x support to the Rh 1 Ni 7 bimetallic interface (Supplementary Fig. 52e ), which is consistent with the electronic structure characterization (Fig. 3d, g ). For the ESR reaction mechanism, the reaction energy barriers for ethanol dehydrogenation and acetaldehyde decomposition were studied through DFT calculations. Based on the calculation results (Supplementary Figs. 53 − 62 , Supplementary Table 8 and Supplementary Note 22 ), the optimal ethanol dehydrogenation path in Ni 8 /TiO 2− x and Rh 1 Ni 7 /TiO 2− x systems follows CH 3 CH 2 OH → CH 3 CH 2 O* → CH 3 CHO* → CH 3 CO*, and then CH 3 CO* undergoes C−C bond breaking to produce CH 3 * and CO, which is consistent with the product distribution and operando characterizations (DRIFTS spectra and pulse experiment). Compared with Ni 8 /TiO 2− x , the energy barriers for ethanol dehydrogenation and C−C bond cleavage decrease from 1.65 and 1.31 eV to 1.03 and 1.17 eV on Rh 1 Ni 7 /TiO 2− x , respectively. For the reaction mechanism of stream reforming of CO (Supplementary Figs. 63 – 72 , Supplementary Table 8 and Supplementary Note 23 ), the potential energy profiles over Rh 1 Ni 7 /TiO 2 -x and Ni 8 /TiO 2- x catalysts are similar and shown in Fig. 5 and Supplementary Fig. 73 , which mainly consists of four steps. Firstly, CO molecule undergoes activation adsorption at the hollow sites (adjacent to two Ni atoms and one Rh atom for Rh 1 Ni 7 /TiO 2 -x ; adjacent to three Ni atoms for Ni 8 /TiO 2 -x ), and then dissociates to form C and O, followed by disproportionation reaction with another CO molecule to generate CO 2 and C species (blue dotted lines in Fig. 5 and Supplementary Fig. 73 ); subsequently, H 2 O molecule experiences activation adsorption at interfacial oxygen vacancy, which dissociates to active hydroxyl and oxygen species (green dotted lines in Fig. 5 and Supplementary Fig. 73 ); afterwards, the hydrogen from H 2 O dissociation binds to the carbon species to generate CH fragment, which is then attacked by active oxygen species to produce the HCOO − intermediate (red dotted lines in Fig. 5 and Supplementary Fig. 73 ); finally, formate undergoes decomposition to produce CO 2 and H 2 (orange lines in Fig. 5 and Supplementary Fig. 73 ). According to the calculation results, the formation of HCOO − intermediate is the rate-determining step with an energy barrier of 2.36 and 2.79 eV on Rh 1 Ni 7 /TiO 2 -x and Ni 8 /TiO 2- x catalysts, respectively. In addition, for the steam reforming processes of CH x , the successive dehydrogenation of methyl occurs firstly on the surface of Ni and RhNi bimetal sites to generate CH fragment (Supplementary Figs. 74 , 75 and Supplementary Note 24 ), followed by a similar process mentioned above for the transform of CH to HCOO − (Supplementary Figs. 67 and 71 ). In contrast, the formate formation from C/CH fragment shows an energy barrier of 2.36 and 2.79 eV on Rh 1 Ni 7 /TiO 2− x and Ni 8 /TiO 2− x catalysts, respectively, much larger than that of ethanol dehydrogenation (1.03 and 1.65 eV) and acetaldehyde decomposition (1.17 and 1.31 eV), indicating that the transformation of CO and CH x is the crucial step, in accordance with the experimental results. Especially, the lower reaction energy barriers on Rh 1 Ni 7 /TiO 2− x relative to Ni 8 /TiO 2− x verify that the ESR reaction is boosted at the bimetal-support interface sites, in well agreement with the catalytic evaluations. Fig. 5: DFT calculation and schematic illustration. Reaction mechanism of stream reforming of CO on the surface of Rh 1 Ni 7 /TiO 2– x . ‘S’ denotes a stable sorption state; ‘TS’ denotes a transition state; ‘ISS’ denotes an intermedia stable state. (Blue, green, red, and orange dotted lines indicate CO disproportionation, H 2 O dissociation, formate generation, and CO 2 desorption, respectively; blue and orange numbers represent adsorption energy and reaction energy barrier, respectively). Full size image In summary, we report a RhNi/TiO 2 catalytic system with well-defined SBMSI towards ESR reaction. The obtained 0.5RhNi/TiO 2 catalyst gives exceptional hydrogen production (H 2 yield: 61.7%) and catalysis stability (300 h) at a relatively low temperature (400 °C). The microscopic fine-structure of RhNi/TiO 2 was studied by STEM, CO-DRIFT, and XAFS, in which the RhNi bimetallic nanoparticle with a reversible TiO 2 coating exhibited a multiple electron transfer pathway at the interfacial active sites (Rh-Ni δ − -O v -Ti 3+ ). A comprehensive investigation including in situ spectroscopic characterizations, operando pulse experiments, kinetics studies, and DFT calculations substantiates that the ESR reaction in the presence of 0.5RhNi/TiO 2 catalyst follows a CO/CH x -mediated reforming process rather than the acetate path. This bimetal-support interface (Rh-Ni δ − -O v -Ti 3+ ) plays a decisive role in the steam reforming of CO and CH x originating from ethanol dissociation, which is involved in the rate-determining step of ESR reaction. The modulated geometric and electronic structure of interfacial active sites resulting from SBMSI reduce the binding ability of species with COO − structure (CO 2 , carbonate, or formate). This facilitates the generation and transformation of formate intermediate from CO/CH x reforming processes, which ensures a prominent hydrogen production rate and catalytic stability. The well-defined SBMSI demonstrated in this work can be extended to other structure-sensitive reactions involving multiple reaction substrates. Chemicals and materials Chemical reagents, including Ni(NO 3 ) 2 ·6H 2 O, Al(NO 3 ) 3 ·9H 2 O, tetrabutyl titanate, anatase, and urea were bought from Aladdin chemical reagent company. RhCl 3 ·3H 2 O was purchased from Beijing HWRK CHEM; absolute ethanol was purchased from Tianjin DaMao chemical reagent factory. The above chemical reagents were used directly without further purification. Quartz sand (SiO 2 , 40−60 mesh) was purchased from Tianjin Guangfu fine chemical research institute, and washed by using concentrated HCl prior to use. Deionized (DI) water with a resistivity of 18.2 MΩ cm was used in all experimental processes. Synthesis of catalysts RhNiTi-LDHs (RhNiTi-layered double hydroxides) precursors were prepared via urea homogeneous precipitation method. Briefly, tetrabutyl titanate (0.013 mol L −1 ), Ni(NO 3 ) 2 ·6H 2 O (0.040 mol L −1 ), and urea (0.500 mol L −1 ) were dissolved in deionized water (150 mL) with vigorous stirring for 8 h at refluxing temperature (95 °C). After 40 min of reaction, a certain amount of RhCl 3 ·3H 2 O aqueous solution (7.6 mg mL −1 ) was slowly dripped into above solution. The resulting precipitate was filtered, washed thoroughly with deionized water until neutral, followed by drying at 80 °C for 12 h to obtain RhNiTi-LDHs. Subsequently, the RhNiTi-MMO (RhNiTi-mixed metal oxide) samples were obtained via calcining the RhNiTi-LDH precursors at 500 °C in air for 4 h followed by cooling to room temperature. Prior to the catalytic reaction, the RhNiTi-MMO samples were treated in a mixture gas (H 2 /N 2 = 1/9; flow rate: 50 mL min −1 ) at 400 °C for 2 h to obtain RhNi/TiO 2 catalysts. The resulting samples with various Rh content are denoted as x RhNi/TiO 2 ( x = 0.1, 0.3, 0.5, 0.8, or 1.0), where the x represents the theoretical mass percentage of Rh (e.g., 0.5RhNi/TiO 2 indicates a 0.5 wt .% Rh in this sample). According to the same method described above, the Rh/Ni and Ni/TiO 2 catalysts were also prepared without the introduction of Ti and Rh, respectively. In addition, the Rh/TiO 2 sample was prepared by traditional impregnation method with 0.5 wt .% Rh loading by using anatase as support. The calcination and reduction conditions are consistent with those of x RhNi/TiO 2 samples. Inductively coupled plasma atomic emission spectroscopy (ICP-AES) is used to determine the chemical composition of these samples, which is close to the feeding ratio (Supplementary Table 1 ). Catalyst characterizations The powder XRD (X-ray diffraction) patterns are recorded on a Rigaku XRD-6000 diffractometer using a nickel-filtered Cu K α radiation source ( λ = 0.15418 nm) at 40 kV and 30 mA with a scanning rate of 8° min −1 and a 2 θ angle ranging from 5° to 80°. Crystalline phases are identified by comparison with the reference data from International Center for Diffraction Data (ICDD) files. The chemical composition of various samples is measured by ICP-AES (Shimadzu ICPS-7500). The specific surface area and pore structure parameters of samples are obtained from N 2 adsorption and desorption isotherms by using a Quantachrome Auosorb-1C-VP analyzer based on the Brunauer-Emmett-Teller (BET) and Barret-Joyner-Halenda (BJH) models. Sample morphology and structure are characterized by scanning electron microscopy (SEM, Zeiss Supra 55) with applied voltage of 20 kV and transmission electron microscopy (TEM, JEOL JEM-2010) with accelerating voltage of 200 kV. Aberration-corrected high-angle annular dark-field scanning transmission electron microscopy (AC-HAADF-STEM) and element energy-dispersive spectroscopy (EDS) mapping images are conducted on a JEOL JEM-ARM200F equipment. The chemical states of sample surface are investigated by using Thermo VG Escalab 250 X-ray photoelectron spectroscopy (XPS) with Al K α as a radiation source at 300 W under UHV (2 × 10 −9 Torr). The sample after treatment was transferred into sample rod in glove box with N 2 atmosphere, and sample charging effects are eliminated by correcting the observed spectra with C 1 s binding energy value of 284.8 eV. Carbon dioxide temperature programmed desorption (CO 2 -TPD), hydrogen temperature programmed desorption (H 2 -TPD), and hydrogen temperature programmed reduction (H 2 -TPR) are carried out on a Micromeritics Chemi-Sorb 2920 instrument equipped with a thermal conductivity detector (TCD). For the CO 2 -TPD, the sample (0.08 g) was firstly pretreated at 400 °C in a H 2 atmosphere for 1 h, followed by purging with He for 0.5 h, and then the temperature was decreased to 50 °C. Subsequently, 5% CO 2 was introduced with He as carrier gas until saturation adsorption. Then, pure He was purged, along with the increase of temperature from 50 to 700 °C (rate: 10 °C min −1 ) for the collection of signals. For the H 2 -TPD, the sample (0.08 g) was firstly pretreated at 400 °C in a H 2 atmosphere for 1 h, followed by purging with Ar for 0.5 h, and then the temperature was decreased to 50 °C. Afterwards, a 5% H 2 was introduced with Ar as carrier gas until a saturation adsorption. The gas was switched to pure Ar, along with the increase of temperature from 50 to 700 °C (rate: 10 °C min −1 ) for signal collection. For the H 2 -TPR, the sample (0.1 g) was firstly pretreated at 250 °C in a Ar atmosphere for 1 h, followed by the decrease of temperature to 50 °C. Then, the gas was switched to a 5% H 2 with Ar as carrier gas. The temperature was increased from 50 to 600 °C with a rate of 10 °C min −1 , and meanwhile the H 2 consumption signal was recorded. In situ diffuse reflectance infrared fourier-transform spectra (in situ DRIFTS) are recorded on a VERTEX 70 BRUKER spectrometer equipped with CaF windows and a mercury-cadmium-telluride (MCT) detector, with a resolution of 4 cm −1 using 100 scans. The catalyst was filled into an in situ reaction cell and pressed into a flat surface. Firstly, the sample was pretreated at 400 °C in a 10% H 2 flow for 1 h followed by purging He for 0.5 h at 400 °C. Prior to the test, the reference baseline was collected; then a switching to CO/CH 4 was performed and the diffuse signals were collected at different time points. Furthermore, H 2 O/H 2 O + CO 2 was introduced by a pulse with N 2 as carrier gas via quantitative loop (1 μL) for signal collection. CO-DRIFT adsorption is carried out at ambiance temperature (20 °C) with CO concentration of 0.5%. For the five-cycle processes of H 2 reduction-O 2 oxidation with 10%H 2 /N 2 and air atmosphere, respectively, the reduction and oxidation were performed for 1.0 h at 400 °C. In situ Raman spectra were recorded on a Renishaw in Via-Reflexm equipped with a laser (532 nm). The catalyst was filled into an in situ reaction cell and pretreated in a 10% H 2 flow at 400 °C for 1 h followed by purging He at 400 °C for 0.5 h. Afterwards, the Raman signals were collected continually during the adsorption of CO and H 2 O/CO 2 . In situ x-ray absorption fine-structure spectra (in situ XAFS) at Ni K-edge and Ti K-edge are performed at the beamline 1W1B of the Beijing Synchrotron Radiation Facility (BSRF), Institute of High Energy Physics (IHEP), Chinese Academy of Sciences (CAS). The 50 mg of different catalysts were filled into an in situ reaction cell and pretreated in a 10% H 2 flow at 400 °C for 1 h followed by purging He at 400 °C for 0.5 h. Afterwards, the signals were collected during the adsorption of CO and H 2 O. Mass spectral analysis of CO and H 2 O pulsing tests are carried out by Micromeritics Chemi-Sorb 2920 instrument equipped with a mass spectrometry detector (MS). Catalytic evaluations for ESR Catalytic performances of as-synthesized samples toward steam reforming of ethanol (ESR) reaction are studied in a fix-bed reactor with a stainless steel tube (interior diameter: 10 mm) at atmospheric pressure. Prior to the catalytic reaction, 0.15 g of catalyst mixed with quartz sand (40−60 mesh, 1.50 g) was pretreated in a gaseous mixture of H 2 and N 2 (1:9, v/v; a total gas flow of 50.0 mL min −1 ) at 400 °C for 2 h, and then cooled to reaction temperature (350 °C and 400 °C) in N 2 atmosphere. The water and ethanol mixture with steam/carbon (S/C) ratio is 3 was injected into the reaction system by using a HPLC pump at a rate of 0.060 mL min −1 . The reactants were evaporated in a preheater (170 °C) with a heating belt to avoid product condensation, followed by mixing with nitrogen gas (50.0 mL min −1 ). The temperature of the whole installation was modulated by a K-type thermocouple. When the reaction was carried out at 350 and 400 °C for 1.5 h, the products were analyzed online by using a gas chromatograph (Shimadzu, GC-17A) with both FID and TCD detectors equipped with TDX-01 and HP-PLOT/Q columns, respectively. Ethanol conversion ( X ), product yield ( Y ), and hydrogen selecticity ( \({S}_{{{{{{{\rm{H}}}}}}}_{2}}\) ) are calculated as following equations. X_EtOH=F_EtOH,in-F_EtOH,out/F_EtOH,in× 100%
 (1) 
    Y_H_2=F_H_2/6×F_EtOH,in× 100%
 (2) 
    Y_C_i=F_C_i× j/2×F_EtOH,in× 100%
 (3) 
    S_H_2=F_H_2/F_H_2+2×F_CH_4+2×__3× 100%
 (4) F EtOH,in/out is the molar flow rate of ethanol at the inlet/outlet of the reactor, respectively. \({F}_{{{{{{{\rm{H}}}}}}}_{2}}\) and \({F}_{{C}_{i}}\) denote the molar flow rate of H 2 and C-containing product at the reactor outlet, respectively, where the j indicates the number of carbon atoms in the latter. The molar flow of acetaldehyde, ethylene, and methane is determined based on FID results. The molar flow of other gas products (H 2 , CO and CO 2 ) in the effluent are measured by TCD results, which are calculated based on Eqs. ( 5 ) and ( 6 ): 
    V_j=V×A_j×y_j^std/A_j^std
 (5) 
    PV=nRT
 (6) where T , P , R, n , and V are the room temperature (K), pressure (Pa), molar gas constant (8.314 J mol −1 K −1 ), molar number, and total volumetric flow of the gas outlet, respectively. A j is the peak area of component j obtained from TCD signal. A std j and y std j are the peak area and the molar fraction of component j in the standard gas mixture, respectively. Reaction dynamics analysis For the measurement of reaction rate of ethanol and acetaldehyde, CO, and CH 4 steam reforming reaction, the quartz sand (SiO 2 , 50−300 mg) and the catalyst sample (5−30 mg) are sieved separately (40−60 mesh) and then physically mixed together before installed into the reactor tube. Reaction conditions for kinetics studies over 0.5RhNi/TiO 2 , Ni/TiO 2 , Rh/Ni, and Rh/TiO 2 catalysts are as follows: liquid feed of ethanol and acetaldehyde at 0.040 mL min −1 , liquid feed of H 2 O at 0.032 mL min −1 , gas flow rate of CO at 50 mL min −1 and CH 4 at 10.0 mL min −1 , CO 2 /H 2 at 10.0 mL min −1 , N 2 carrier at 50 mL min −1 , reaction temperature: 240−400 °C, time on stream: 0.5 h. For the determination of reaction order of ethanol dehydrogenation and acetaldehyde decomposition, the initial partial pressure of ethanol and acetaldehyde are 7−39 kPa and 4−15 kPa, respectively. For the determination of the reaction order of CH 4 steam reforming, the initial partial pressure of CH 4 is 4−12 kPa. For the determination of the reaction order of CO steam reforming, the initial partial pressure of H 2 O, CO, CO 2 , and H 2 is tuned within 20−40 kPa, 4−17 kPa, 3−13 kPa, and 4−23 kPa, respectively. Computational details Density functional theory (DFT) calculations are performed in Vienna ab initio simulation package (VASP) with the generalized gradient approximation (GGA) using the Perdew-Burke-Ernzerhof (PBE) functional [46] . The projected augmented wave (PAW) potentials are used to describe the ionic cores, and valence electrons are also considered using a plane wave basis set with a kinetic energy cutoff of 400 eV [47] . Geometry optimizations are performed with the force convergency smaller than 0.05 eV A −1 , where the same convergency is applied for the location of transition states by the constrained optimizations. The original bulk structure is optimized before the construction of surfaces with the Monkhorst-Pack k-point of 3 × 3 × 1. The TiO 2 (110) surface with 24 Ti and 48 O atoms is applied with half of the atoms at the bottom fixed in all the calculations. A Ni 8 cluster with 8 Ni atoms is placed on the TiO 2 (110) surface to describe the interface of Ni/TiO 2 . According to the STEM results, one Ni atom is then replaced by one Rh atom on Ni 8 surface to build the RhNi/TiO 2 interface structure. A Monkhorst-Pack k-point 3 × 3 × 1 is applied for all the calculations on surfaces. In addition, the effect from the Hubbard U corrections is considered beyond the accuracy of DFT calculations of GGA, where U value (employed as U-J) of 3.5 is applied for Ti, Ni, and Rh. Transition state (TS) searches are performed at the same theoretical level with the CI-NEB method. All the models are the most stable structure obtained through optimization and screening. The formation energy ( FE O v ) is used in analyzing oxygen vacancy formation (O v ), defined as 
    FE_Ov=E_vo-slab+E_o-gas-E_slab
 (7) where E vo-slab , E o-gas , and E slab are the total energies for the oxygen vacancy slab, the oxygen atom in the gas phase, and the clean surface, respectively. The adsorption energy ( E ads ) is calculated as 
    E_ads=E_total-(E_slab+E_g)
 (8) where E total is the total energy after adsorption; E slab is the energy of the clean slab before adsorption, and E g is the energy of the free adsorbate in the gas phase. The energy barrier ( E a ) is obtained from the electronic energy difference between the transition state ( E TS ) and its corresponding initial state ( E IS ), which is calculated by 
    E_a=E_TS-E_IS
 (9) In this work, a Ni 7 Rh 1 /TiO 2– x model is applied for calculation, in which Ni 7 Rh 1 cluster is supported on the TiO 2 (110) surface with oxygen vacancy. Before the calculations, the model of Ni 7 Rh 1 /TiO 2– x is optimized. The lattice parameters of TiO 2 support are: a = b = 3.79 Å, c = 9.56 Å, α = β = γ = 90° (body-centered tetragonal) with a p(2 × 2) supercell.